Optical transmission enhacement through chemically tuned two-dimensional bismuth chalcogenide nanoplates Layer-structured two-dimensional nanomaterials are a family of materials with strong covalent bonding within layers and weak van der Waals interaction between layers, whose vertical thickness can be thinned down to few nanometer and even single atomic layer. Bismuth chalcogenides are examples of such two-dimensional materials. Here, we present our discovery of significant enhancement of light transmission through thin nanoplates of layered bismuth chalcogenides by intercalation of copper atoms, which is on the contrary to most bulk materials in which doping reduces the light transmission. This surprising behaviour results from two mechanisms: chemical tuning effect of substantial reduction of material absorption after intercalation and nanophotonic effect of zero-wave anti-reflection unique to ultra-small thickness of nanoplates. We demonstrate that the synergy of these two effects in two-dimensional nanostructures can be exploited for various optoelectronic applications including transparent electrode. The intercalation mechanism allows potential dynamic tuning capability. Beyond graphene [1] , [2] , [3] , [4] , [5] , [6] , two-dimensional (2D) materials like boron nitride [7] , [8] and a variety of metal chalcogenides [9] , [10] , [11] , [12] , [13] have been shown to host a variety of interesting physical and chemical properties [14] , [15] , [16] , [17] , [18] , [19] , [20] . As members of this 2D material family, Bi 2 E 3 (E=Se, Te) have been extensively studied for thermoelectrics [21] , [22] , [23] . More recently, they have been discovered to be topological insulators and have caused a great research attention on these materials [14] , [15] , [16] , [17] . These chalcogenides exhibit a layered, rhombohedral crystal structure as shown in Fig. 1a . Each layer consists of five covalently bonded atomic planes, E-Bi-E-Bi-E, known as a quintuple layer. These quintuple layers are bonded together via van der Waals interaction to form the Bi 2 E 3 crystal. Each quintuple layer has a thickness of about 1 nm. Copper (Cu) intercalated Bi 2 Se 3 has been found to show superconducting behaviour at low temperature [24] . Recently, we and others have demonstrated the growth of Bi 2 E 3 nanoribbons and nanoplates with thickness down to 3 nm for studying the physics of topological insulator states [17] , [25] . Chemical species can be inserted between layered materials via a process known as intercalation [26] . 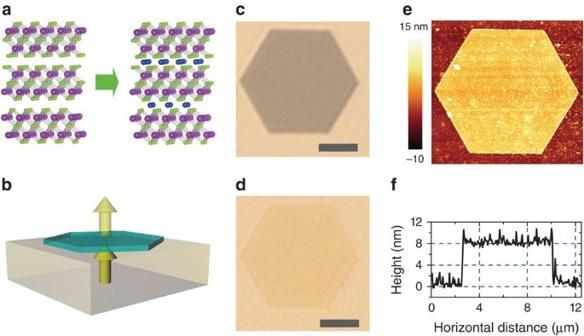Figure 1: Cu intercalation induced transparency in bismuth chalcogenide nanoplates. (a) Crystal structures of the Bi2E32D materials. Purple, Bi; green, Se; blue, Cu. Through intercalation processes, Cu atoms can be inserted into the van der Waals gaps between the quintuple layers. (b) Schematic of light transmission through a bismuth chalcogenide nanoplate on top of transparent substrate. The yellow arrows show the propagation direction of light. (c) Optical transmission image of an 8-nm thick pristine Bi2Se3nanoplate on glass substrate. Scale bar, 4 μm. (d) Image of the same nanoplate as incafter Cu intercalation. (e) Atomic force microscopy (AFM) image of the same plate as inc. (f) Line profile across the AFM image ine, which gives a clear reading of the nanoplate thickness. Figure 1: Cu intercalation induced transparency in bismuth chalcogenide nanoplates. ( a ) Crystal structures of the Bi 2 E 3 2D materials. Purple, Bi; green, Se; blue, Cu. Through intercalation processes, Cu atoms can be inserted into the van der Waals gaps between the quintuple layers. ( b ) Schematic of light transmission through a bismuth chalcogenide nanoplate on top of transparent substrate. The yellow arrows show the propagation direction of light. ( c ) Optical transmission image of an 8-nm thick pristine Bi 2 Se 3 nanoplate on glass substrate. Scale bar, 4 μm. ( d ) Image of the same nanoplate as in c after Cu intercalation. ( e ) Atomic force microscopy (AFM) image of the same plate as in c . ( f ) Line profile across the AFM image in e , which gives a clear reading of the nanoplate thickness. Full size image In our previous work, we developed a novel chemical approach of zero-valent metal atom intercalation into these nanostructures and demonstrated that a variety of metal atoms can be intercalated [27] , [28] , which is different from the historical development of positively charged metal ion intercalation. Very high concentration of Cu atom interaction (up to 60%) has been controllably demonstrated [27] . As material optical property is strongly dependent on its electronic structure, it is intriguing to tune the optical properties of Bi 2 E 3 with this novel intercalation approach. In the following, we report counter-intuitive optical transparency of Bi 2 E 3 nanoplates induced by Cu intercalation. Simultaneous enhancement of optical transmission and electrical conductivity will enable various applications of these materials. Material preparation and characterization Bi 2 Se 3 nanoplates from a few to a few tens of nanometer thick, with a lateral dimension around a few tens of micrometres are synthesized using solvothermal method [29] . Cu atoms are intercalated into Bi 2 Se 3 nanoplate following our previous procedures [27] , [28] . The amount of Cu intercalants can be controlled by varying the reaction time from several minutes to a few hours. In this study, the atomic concentration of Cu we intercalated into the nanoplates ranges from 0 to around 20%. Optical transmission measurements ( Fig. 1b ) of individual plates before and after intercalation were conducted to compare the changes due to the Cu intercalation. Figure 1c,d provides transmission optical images of the same Bi 2 Se 3 nanoplate with thickness of 8 nm before and after 1 h of Cu intercalation, respectively. The thickness of the plate before intercalation is determined by the atomic force microscopy as shown in Fig. 1e,f . There is no noticeable change in nanoplate thickness after Cu intercalation ( Supplementary Fig. 1 ). Substantial transmission change can be observed directly from the images since the nanoplate looks much brighter after intercalation under the same illumination condition. As a control, we also treated Bi 2 Se 3 samples in the same solvent, but without the Cu salt. There is no observable change in their optical transmission, suggesting that Cu intercalation instead of the solvent makes the nanoplate much more transparent. To confirm the Cu intercalation into the nanoplate, we have carried out transmission electron microscopy (TEM) study. 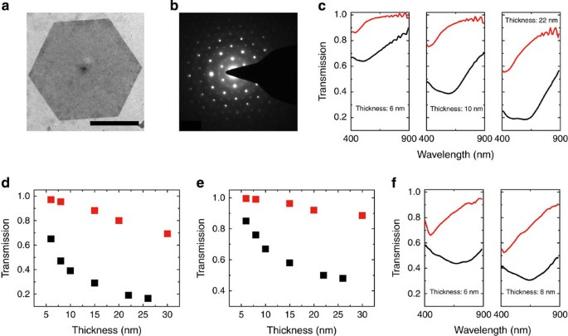Figure 2: TEM and optical characterizations of bismuth chalcogenide nanoplates. (a) TEM image of a Bi2Se3nanoplate. Scale bar, 2 μm. (b) Electron diffraction pattern of a Bi2Se3nanoplate intercalated with ~22 at% Cu. There is no difference compared with diffraction patterns for pristine nanoplates. (c) Optical transmission spectra of Bi2Se3nanoplates with various thicknesses before (black) and after (red) Cu intercalations. Thickness dependence of nanplates’ optical transmissions is shown at 550 nm (d) and 850 nm (e) wavelengths, respectively. Black squares, before Cu intercalation; red squares, after Cu intercalation. (f) Optical transmission spectra of two Bi2Te3nanoplates with thicknesses of 6 and 8 nm. Their transmission spectra after Cu intercalation are also shown. Figure 2a is a TEM image of a Bi 2 Se 3 nanoplate. Energy dispersive X-ray spectroscopy measurements are carried out in TEM to determine the ratio of Bi, Se and Cu after the intercalation ( Supplementary Fig. 2 ). Measurements of samples with various amounts of Cu intercalants show that the stoichiometric ratio between Bi and Se remained the same as before intercalation. X-ray diffraction results in ref. 27 have shown that up to 20–30% Cu intercalation causes very small lattice expansion (<1%). Here electron diffraction results ( Fig. 2b ) also show that the crystal structure of the nanoplates did not change with 22 at% intercalated Cu, which is evident that the host crystal lattice was not distorted by the added Cu atoms. The zero-valent nature of Cu intercalants have been clearly demonstrated in our previous studies [27] . Figure 2: TEM and optical characterizations of bismuth chalcogenide nanoplates. ( a ) TEM image of a Bi 2 Se 3 nanoplate. Scale bar, 2 μm. ( b ) Electron diffraction pattern of a Bi 2 Se 3 nanoplate intercalated with ~22 at% Cu. There is no difference compared with diffraction patterns for pristine nanoplates. ( c ) Optical transmission spectra of Bi 2 Se 3 nanoplates with various thicknesses before (black) and after (red) Cu intercalations. Thickness dependence of nanplates’ optical transmissions is shown at 550 nm ( d ) and 850 nm ( e ) wavelengths, respectively. Black squares, before Cu intercalation; red squares, after Cu intercalation. ( f ) Optical transmission spectra of two Bi 2 Te 3 nanoplates with thicknesses of 6 and 8 nm. Their transmission spectra after Cu intercalation are also shown. Full size image To further study the behaviour of such an optical property transition, spectral measurements were carried out to characterize the same individual nanoplates before and after Cu intercalation. The confocal measurement was conducted on single nanoplates to ensure that the detected light is from the nanoplate sample only and not mixed with signals from other area of substrate. The confocal mechanism allows the collection of light from a spot approaching the diffraction limit (<~1 μm), which is much smaller than the lateral size of nanoplates (typically 5–20 μm). All optical transmission data are normalized to the transmission of bare glass substrate. Figure 2c shows the transmission spectra of Bi 2 Se 3 nanoplates, with 6, 10, 22 nm thicknesses before (black curves) and after (red curves) 1 h of Cu intercalation. Clear thickness dependence of the transmission spectra allows us to compute the optical properties of both intrinsic and Cu-intercalated materials as we will show in the next section. Figure 2d,e plots the transmission versus nanoplate thickness for two different optical wavelengths: 550 nm (visible) and 850 nm (near-IR), respectively. Before Cu intercalation, the optical transmission is relatively low for all thicknesses of nanoplates. In contrast, the transmission increases dramatically for all thicknesses and for all the wavelengths (400–900 nm) measured after Cu interaction. For example, for the bare nanoplates with a thickness of 22 nm, the transmission in visible frequency is only about 20%. After Cu intercalation, the transmission is boosted to over 70% in most part of the visible-near-IR range. Thin plates <10 nm thick become highly transparent (>95%) after Cu intercalation. Moreover, the transmission in long wavelength range is usually more than that in the short one ( Fig. 2c–e ). Such a feature is preserved even after Cu intercalation, which is a characteristic of the mechanism we provided in the next section. In addition to Bi 2 Se 3 nanoplates, similar optical transmission enhancement after Cu intercalation has also been observed in Bi 2 Te 3 nanoplates, as shown in Fig. 2f . The behaviour of transmission enhancement is actually caused by combined optical and electronic effects. Below we provide experimental evidence that explains the mechanism of the anomalous reduction of absorption and formulate the light transmission through the nanoplates. The nanoplates’ ultra-small thicknesses, which are much less than the wavelength of light, lead to very unique optical reflectance responses. Theoretical analysis Substantial reduction of absorption at optical frequencies can be attributed to an ultra-large Burstein–Moss shift of the bandgap caused by the large amount of free electrons introduced to the material via intercalation of Cu atoms. For degenerately doped semiconductors, increased free electron density will effectively elevate the Fermi level into the conduction band. Therefore, electrons from valence band cannot be excited to the bottom level of the conduction band, but the first unoccupied level above the Fermi level, that is, the effective bandgap has been increased, as shown in Fig. 3a . Compared with the degenerate doping (a few percent or less) of usual semiconductors, the Cu intercalation doping concentration (22%) in 2D materials is much more substantial. The Burstein–Moss shift is expected to be much larger in 2D nanoplates. 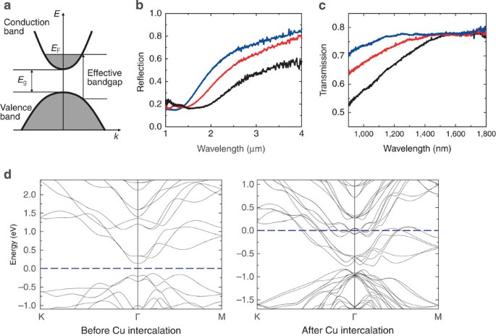Figure 3: Optical bandgap widening induced by increased free electron density. (a) Schematic showing the Burstein–Moss shift induced by the increased free electron density.EF, Fermi level,Eg, width of the intrinsic bandgap. (b) Optical reflection spectra of thick Bi2Se3ribbons showing the blue shift of plasma edge after different time of Cu intercalation. black, 30 min; red, 45 min; blue, 1 h of intercalation. (c) Transmission spectra of the same Bi2Se3nanoplate (20-nm thick) showing the widening of optical bandgap after different time of Cu intercalation. Black, 15 min; red, 25 min; blue, 35 min of intercalation. (d) Bi2Se3band structure before and after Cu intercalation, based on first-principles density functional theory calculations. The blue dashed lines indicate the positions of Fermi levels. Figure 3: Optical bandgap widening induced by increased free electron density. ( a ) Schematic showing the Burstein–Moss shift induced by the increased free electron density. E F , Fermi level, E g , width of the intrinsic bandgap. ( b ) Optical reflection spectra of thick Bi 2 Se 3 ribbons showing the blue shift of plasma edge after different time of Cu intercalation. black, 30 min; red, 45 min; blue, 1 h of intercalation. ( c ) Transmission spectra of the same Bi 2 Se 3 nanoplate (20-nm thick) showing the widening of optical bandgap after different time of Cu intercalation. Black, 15 min; red, 25 min; blue, 35 min of intercalation. ( d ) Bi 2 Se 3 band structure before and after Cu intercalation, based on first-principles density functional theory calculations. The blue dashed lines indicate the positions of Fermi levels. Full size image A substantial blue shift of plasma edge provided direct evidence of the increasing amount of free electron associated with Cu intercalation. The free electron effect on electrical permittivity can be described by the Drude model [30] . where is the angular frequency of plasma oscillations, which is directly dependent on the free carrier concentration N , m * is the effective mass of electrons, ε ∞ is the high-frequency dielectric constant and Γ is the damping constant of the free electron plasma. As the frequency of light decreases, real part of the permittivity decreases from positive to large negative values, which provides clear signatures in the reflection of the material. A minimum in reflection is expected close to where the permittivity switches sign from positive to negative [31] , [32] . It is then followed by a substantial increase in reflection. Such plasma edge behaviour is observed in the reflection spectra measured on Cu-intercalated Bi 2 Se 3 ribbons, as shown in the reflection measurements in Fig. 3b . As more and more Cu atoms are intercalated, the plasma edge of the material moves toward shorter wavelengths, since the plasma frequency has a blue shift associated with the increasing concentration of free electrons. Our observation is also consistent with the finding that Cu atoms added to interstitial sites provide free electrons to Bi 2 Se 3 system [31] . The reflection measurement results can be fitted with the Drude model to obtain the concentration of free electrons in the materials ( Supplementary Fig. 3 ), which yields an extremely high free electron concentration on the order of 10 21 cm −3 . It is a great advantage of the 2D material systems that a large number of foreign atoms can be added to the van der Waals gap without damaging the host crystal lattice. Associated with the addition of a plethora of free electrons are the elevation of Fermi level and the increase of effective bandgap, which can be observed through absorption edge measurement. As shown in Fig. 3c , the effective bandgap gradually increases as more Cu atoms are intercalated. With 2-h intercalation of Cu, we observed that the effective optical bandgap has been widened to around 1.1 eV, which is substantial compared with the initial small gap around 0.3–0.5 eV. When the bandgap approaches higher energy scales, material absorption at optical frequencies is substantially decreased. First-principles simulations provide us evidence of the substantial Fermi level shift. As shown in the calculated electronic structure before and after intercalation ( Fig. 3d ), the Fermi level lies in the bandgap for intrinsic Bi 2 Se 3 , but gets deep into the conduction band with Cu intercalation. The calculated separation between Fermi level and the top of the valence band for intercalated samples reaches ~1 eV, consistent with our experimental observation. Unlike previous studies [33] , [34] with small shifts in a very narrow energy range by regular doping, the ultra-large shift due to Cu intercalation here enables dramatic optical property change over a large wavelength range, thus makes such a material system suitable for applications that require substantial optical property tuning. 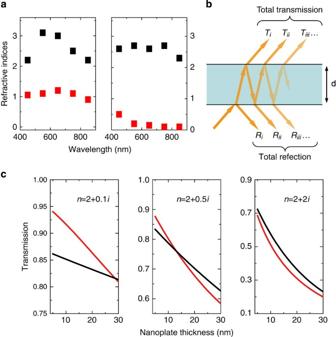Figure 4: Optical loss reduction and optical interference in nanoplates. (a) Refractive indices of Bi2Se3before and after Cu intercalation, calculated from the experimental data. Black squares are the real parts and red squares are the imaginary parts. (b) Schematic of multiple reflection of light inside a thin film (light blue part with thicknessd). Arrows show the propagation directions of light waves.Ti, Tii, … andRi, Rii, … are different orders of transmission and reflection. Interference of the waves may modify the actual transmission and reflection. (c) Calculated transmission of films at 550 nm wavelength showing the effect of zero-wave anti-reflection for low-absorption material. The refractive indices for the three cases shown in different panels are:n=2+0.1i, 2+0.5iand 2+2i, respectively. Black curves, 0th-order transmission (no multiple reflection and interference effect). Red curves, total transmission with interference effect. Figure 4a shows the refractive indices obtained from the experimental data. The transmission of light through the nanoplates has a direct dependence on their thicknesses; therefore the optical properties of the material can be calculated based on transmission data through nanoplates with different thicknesses. Substantial reduction of the imaginary parts of the material’s refractive index after Cu intercalation, as shown in Fig. 4a , indicates the decrease of light absorption. When such an optical property change happens to nanoplates and potentially ultra-thin films, it is further magnified by the interference effect, which is referred to as zero-wave anti-reflection effect here. Considering a light beam passing through a nanoplate with thickness d , it experiences multiple reflections at the top and bottom surfaces of the nanoplates ( Fig. 4b ). For normally incident light, the total transmitted light can be expressed as follows: Figure 4: Optical loss reduction and optical interference in nanoplates. ( a ) Refractive indices of Bi 2 Se 3 before and after Cu intercalation, calculated from the experimental data. Black squares are the real parts and red squares are the imaginary parts. ( b ) Schematic of multiple reflection of light inside a thin film (light blue part with thickness d ). Arrows show the propagation directions of light waves. T i , T ii , … and R i , R ii , … are different orders of transmission and reflection. Interference of the waves may modify the actual transmission and reflection. ( c ) Calculated transmission of films at 550 nm wavelength showing the effect of zero-wave anti-reflection for low-absorption material. The refractive indices for the three cases shown in different panels are: n =2+0.1 i , 2+0.5 i and 2+2 i , respectively. Black curves, 0th-order transmission (no multiple reflection and interference effect). Red curves, total transmission with interference effect. Full size image where E t is the electric field amplitude of the transmitted light, E 0 is that of the incident light and k is the wavevector of light inside the nanoplate. t 1 and t 2 are the transmission coefficients at the first and second interface, respectively [35] . r 1 and r 2 are the reflection coefficients at those interfaces. where n 1 , n 2 and n 3 are the refractive indices of the substrate, nanoplate and air, respectively. Unlike the widely used quarter-wave anti-reflection coatings for many optical devices, here reflections from top and bottom surfaces of bismuth chalcogenide nanoplates have different phase relations due to the refractive index with a non-zero imaginary part and a real part larger than the surrounding media. Figure 4c is a comparison between materials with different absorption capabilities. In the low-absorption case, r 1 and r 2 have opposite signs ( π phase difference). Different orders of transmissions interfere constructively in the thin-film limit, as shown in equation (1). Reflection is suppressed. However, such anti-reflection interference will be damaged when strong absorption is present, because further phase shift is caused by the complex refractive index. The phase change of reflections at both interfaces can be obtained using equation (4), given the refractive indices at different wavelengths. The phase difference between r 1 and r 2 is away from π . Reflection may even be enhanced as shown in the right panel of Fig. 4c . Therefore, absorption reduction adjusts the phase shifts of the reflections and leads to a more constructive interference condition for optical transmissions through the nanoplates. Substantial reduction in the imaginary part of the refractive index leads to two effects, both of which enhance the transmission of the nanoplates: the reduction of direct absorption and reflection phase shifts at both interfaces that helps the interferential anti-reflection effect as described above. The synergy of these two effects makes the Cu intercalation-induced transparency more substantial. Such an optical transmission enhancement together with metallic Cu intercalation opens up exciting opportunities for applications such as transparent electrodes. Due to the ultra-high carrier density provided by the Cu intercalants, the Bismuth chalcogenide nanoplates also exhibit very good electrical conductivity even at small thicknesses. Sheet resistance before and after Cu intercalation was measured on single Bi 2 Se 3 nanoplate devices, fabricated by using the standard e-beam lithography and thermally evaporated Cr/Au contacts. 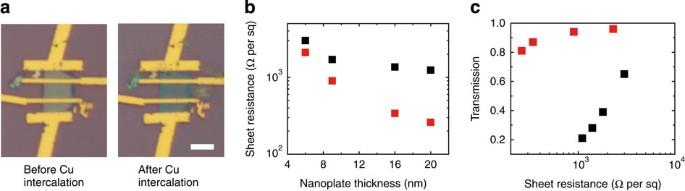Figure 5: Enhanced electrical conductivity with Cu intercalation. (a) A Bi2Se3nanoplate-based four-point probe measurement device on silicon substrate, with gold electrodes. Scale bar, 5 μm. (b) Sheet resistances are substantially reduced for Bi2Se3nanoplates with different thicknesses after Cu intercalation. (c) Transmission-sheet resistance map showing the enhancement of both transparency and conductivity of the nanoplates. Figure 5a shows that contacts remain intact after intercalation and the plate colour changes. As shown in Fig. 5b , the sheet resistances decreased dramatically after intercalation by two to fivefolds. The improvement of both conductivity and transparency is desirable for transparent electrodes. Figure 5c provides the transmission-sheet resistance map of different samples. Materials with properties in the upper left corner of the map are good candidates for transparent electrodes. Our results suggest that Cu intercalation leads to both increased transparency and high conductance. Such a performance is potentially interesting for touch screen applications. Figure 5: Enhanced electrical conductivity with Cu intercalation. ( a ) A Bi 2 Se 3 nanoplate-based four-point probe measurement device on silicon substrate, with gold electrodes. Scale bar, 5 μm. ( b ) Sheet resistances are substantially reduced for Bi 2 Se 3 nanoplates with different thicknesses after Cu intercalation. ( c ) Transmission-sheet resistance map showing the enhancement of both transparency and conductivity of the nanoplates. Full size image The mechanism described here does not have a strong dependence on the host material as long as carrier density can be greatly changed by metal intercalants. Therefore besides Bi 2 Se 3 and Bi 2 Te 3 , similar behaviour may be found in various other 2D material systems through intercalation approaches. And it is particularly attractive to be able to manipulate the positions of the absorption edge and the plasma edge, by controlling the amount of Cu intercalated. In this way, we can flexibly tune the transmission band over a wide range of frequencies from visible to infrared. The high transmittance in infrared further extends the tuning range beyond the wavelength of 1.6 μm where existing transparent conducting oxide materials do not have a good transmittance. Moreover, as extensively studied in electrochemistry [26] , intercalation and deintercalation in 2D materials can be achieved by electrochemical methods; therefore dynamic tuning of optical properties in a large scale is possible. For example, electrochemical control of photoluminescence in 2D MoS 2 nano flakes based on intercalation and deintercalation processes have been studied recently [36] . The 2D-layered structure of bismuth chalcogenide materials enables the formation of ultra-thin flat plate and intercalation of large amount of metal atoms. By intercalating Cu atoms into Bi 2 Se 3 and Bi 2 Te 3 nanoplates, we are able to tune the optical and electrical behaviour of such materials. Synergetic effect from chemical tuning and zero-wave anti-reflection leads to substantial optical transmission improvement in those nanoplates, together with enhanced electrical conductivity. The great potential in tuning the physical and chemical properties of such materials will lead to various applications including transparent electrodes, tunable optoelectronic devices. Solvothermal synthesis of bismuth selenide nanoplates High-purity polyvinylpyrrolidone (PVP) was first dissolved in ethylene glycol. A mixture of Bi 2 O 3 powder, selenium powder and ethylenediamine tetraacetic acid (EDTA) powder was added to the solution and thoroughly stirred to form a suspension. The suspension was then sealed in a steel autoclave and kept at a temperature in the range of 180–220 °C for 24 h. The lateral dimension of the single-crystalline products was observed to be up to a few tens of micrometres and their thicknesses were typically several to a few tens of nanometres. Vapour phase growth of bismuth telluride nanoplates A purity of 99.999% Bi 2 Te 3 powder was heated up in a tube furnace to around 500 °C and transformed to vapour phase. Ar gas flow was applied to the vacuum tube furnace and carried the Bi 2 Te 3 vapour to the end of the furnace where a substrate was placed. As the temperature around the end of the furnace was much lower than the centre part, the molecules in the vapour started to deposit on the substrate and formed ultra-thin triangular or hexagonal nanoplates. Quartz substrate was used to allow the measurement of the transparency of Bi 2 Te 3 nanoplates. Intercalation of Cu into Bi 2 Se 3 and Bi 2 Te 3 nanoplates For the consistency of optical measurements, nanoplates were first drop-casted on a glass slide. After drying, they were added into a mixture of 5 ml butanol with 3 mg Tetrakis(acetonitrile)Cu (i) Hexafluorophosphate ([Cu(CH 3 CN) 4 ]PF 6 ) from Sigma-Aldrich and heated to around 55 °C (ref. 27 ). The amount of Cu intercalated is controlled by the reaction time. Nanoplate optical transmission and reflection measurements Bi 2 Se 3 nanoplate suspension was first drop-casted on glass substrate and their optical transmissions were measured using a Nikon C1 confocal microscope. The spectra were analysed using the Princeton Instruments Acton SpectraPro 2300i spectrograph and Pixis 1024 Si CCD detector. Reflection spectra were measured using Bruker Hyperion 2000 infrared microscope and IFS-125/HR Fourier transform infrared spectrometer. Numerical simulations First-principles density functional theory calculations are performed to obtain the electronic band structure of the undoped Bi 2 Se 3 and the Cu-intercalated Bi 2 Se 3 for both bulk ( Fig. 3d ) and a few quintuple layer cases ( Supplementary Figs 4,5 ). We use the Hohenberg–Kohn density functional theory with the generalized-gradient approximation and the projector augmented-wave method as implemented in Vienna Ab initio Simulation Package (VASP). Intercalated Cu atoms are at the tetrahedral sites in the van der Waals gap of Bi 2 Se 3 , which lead to the lowest energy configuration. Spin-orbit coupling effect is included in the band structure calculations. The band structures are plotted along the high-symmetry directions K-Γ-M in the reciprocal space of the hexagonal lattice. How to cite this article: Yao, J. et al . Optical transmission enhacement through chemically tuned two-dimensional bismuth chalcogenide nanoplates. Nat. Commun. 5:5670 doi: 10.1038/ncomms6670 (2014).